High-quality electron beams from a helical inverse free-electron laser accelerator Compact, table-top sized accelerators are key to improving access to high-quality beams for use in industry, medicine and academic research. Among laser-based accelerating schemes, the inverse free-electron laser (IFEL) enjoys unique advantages. By using an undulator magnetic field in combination with a laser, GeV m −1 gradients may be sustained over metre-scale distances using laser intensities several orders of magnitude less than those used in laser wake-field accelerators. Here we show for the first time the capture and high-gradient acceleration of monoenergetic electron beams from a helical IFEL. Using a modest intensity (~10 13 W cm −2 ) laser pulse and strongly tapered 0.5 m long undulator, we demonstrate >100 MV m −1 accelerating gradient, >50 MeV energy gain and excellent output beam quality. Our results pave the way towards compact, tunable GeV IFEL accelerators for applications such as driving soft X-ray free-electron lasers and producing γ-rays by inverse Compton scattering. The free-electron laser (FEL) interaction [1] , [2] is one of the most efficient mechanisms of transferring energy from a relativistic electron beam to a radiation pulse, and as such forms the physical basis of the revolutionary successes of fourth generation coherent X-ray light sources [3] , [4] . Coupling between transverse electromagnetic waves and relativistic electron motion is made possible in the FEL by the presence of the undulator magnetic field that bends the electron trajectories, enabling the energy exchange. Synchronous energy transfer is achieved if the electrons’ oscillations fall behind laser wavefronts by an integer number of wavelengths for each undulation period (resonant condition). In FELs, the electrons on average lose energy to the electromagnetic wave as they propagate through the undulator field. The same mechanism can be employed in reverse to enable laser-driven acceleration of particles by extracting energy from a high-power laser to accelerate a relativistic electron beam at high gradients [5] , [6] . To achieve large energy gains in this case, the inverse FEL (IFEL)/FEL resonant condition can be maintained over metre-scale distances by appropriately tapering the undulator magnetic field and period. The gradients available in the IFEL accelerator approach the GeV m −1 level with current laser and undulator techonolgy. The IFEL enjoys unique advantages over other advanced accelerator schemes. The IFEL does not require any medium (plasma or dielectric) or boundaries close to the interaction, allowing for efficient coupling as the energy from the laser is directly transferred into electron kinetic energy rather than dissipating in a medium. As a far-field vacuum acceleration scheme, nearly plane wave electromagnetic radiation can be used to accelerate particles, removing all issues related to small transverse acceptance or strong focusing in optical frequency or plasma-based accelerating structures. The transverse beam size can therefore be relatively large (many laser wavelengths across), which, in addition to the absence of nearby structures, strongly mitigates collective effects such as space charge or wakefields [7] . Furthermore, the IFEL has an advantage in terms of achievable gradient for a given laser intensity. The rate of change in energy for an IFEL is proportional to the product of the laser and undulator vector potential amplitudes and given by d γ /d z = kK 1 K JJ sin φ/2 γ , where γ is the Lorentz factor, φ = k w z + kz −ω t is the ponderomotive phase—that is, the phase of particles in the cosine-like potential formed by the combined action of the laser and undulator fields. K 1 = eE 1 / kmc 2 and K = eB w / k w mc are the laser and undulator normalized vector potential amplitudes, E 1 and B w are the laser electric and undulator magnetic field amplitudes, and k and k w are the laser and undulator wavenumbers. We assume K 1 ≪ K in this paper. JJ is an undulator coupling factor of order unity, which is expressed as JJ= J 0 (χ)− J 1 (χ) with χ −1 =2(1+ K −2 ) for planar and as JJ=2 for helical undulators. As the undulator parameter K can be easily made larger than unity using few-cm long periods and 0.5 T-level fields, impressive gradients can be sustained even at non-relativistic laser intensities. To draw a comparison, laser wake field accelerators (LWFAs) present a characteristic dependence of the accelerating wave amplitude as and have only demonstrated significant energy gain with relativistic (that is, K 1 >1) laser intensities [8] . Although the practical limit of the final IFEL energy is in the tens of GeV range because of synchrotron radiation losses, the IFEL is perfectly suited as a driver for 1–2 GeV electron beam applications like soft X-ray FELs and the production of γ-rays by inverse Compton scattering [9] . To give a historical context for our current results, we review previous high-energy IFEL experiments. The BNL STELLA experiment [10] staged a microbuncher and gap-tapered, planar undulator to produce monoenergetic electron beams with energy gain of up to 9 MeV. This experiment took advantage of one of the characteristics of the IFEL output beam to be composed by a sequence of microbunches phase-locked to the drive laser frequency. The UCLA Neptune IFEL experiment [11] achieved 20 MeV energy gain and 70 MeV m −1 peak gradient with a period and magnetic field tapered undulator and strongly focused high-power CO 2 laser. To date, IFEL accelerators have used planar undulators to couple electronic motion to laser fields. In this geometry, the electron velocity component parallel to the laser electric field is periodically reduced to zero, effectively halting the energy transfer twice per period as illustrated in Supplementary Fig. 1 . Employing a helical undulator magnetic field induces a helical motion for the electrons, which provides continuous energy transfer with a circularly polarized laser of the same handedness. To quantify, the IFEL coupling strength is proportional to the Bessel factor JJ. For planar undulators, this term approaches unity for small K and approximately 0.7 for large K , whereas for helical undulators, JJ=2, more than doubling the gradient. In this paper, we report the first demonstration of a helical IFEL accelerator to achieve 54 MeV energy gain and 100 MeV m −1 average accelerating gradient by the UCLA-BNL helical IFEL collaboration at the Brookhaven Accelerator Test Facility (ATF) [12] . The 54-cm long IFEL undulator used in the experiment is the first ever strongly tapered undulator with a helical geometry. By carefully tuning the undulator tapering, we have also demonstrated capture of a large fraction (~30%) of the injected electron beam and monoenergetic acceleration with a final energy spread of the captured beam smaller than 1.8%. The emittance of the accelerated beam is also measured and found in agreement with three-dimensional simulations. The gradients achieved exceed that of conventional radiofrequency (RF) accelerators and are achieved with laser intensities of order 10 13 W cm −2 —nearly five orders of magnitude lower than those used in LWFA experiments. 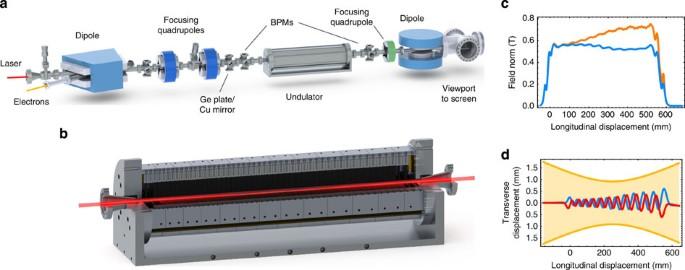Figure 1: Layout of the helical IFEL experiment at Brookhaven ATF. (a) Beamline layout with helical undulator installed just upstream of a wide-angle energy spectrometer shown at the far right. The CO2laser beam is injected from the far left-hand side of the beamline while the electron beam is kicked onto the beamline from the left-most dipole. (b) Cutaway and zoom of the strongly tapered helical undulator. (c) Magnitude of the undulator fields for the high-gradient (orange) and reduced field, high-efficiency (blue) undulator tapering configurations. (d) Electron beam trajectories for the high-gradient undulator configuration inferred from the second integrals of the measured fields assuming constant 52 MeV input electron beam energy. The trajectories are superimposed on top of a plot of the 1/e2CO2laser spot size as measured by scanning a pyroelectric camera near the waist. Experimental setup Figure 1a shows the experimental layout of the interaction area. A 52-MeV input energy electron beam and terawatt (TW)-class circularly polarized 10.3 μm wavelength CO 2 laser [13] are co-propagated in the 54-cm long first ever strongly tapered helical undulator (see Methods). The unique magnetic field configuration is obtained using two perpendicularly oriented permanent-magnet Halbach undulators [14] with constant gap of 15 mm and shifted in phase by π/4 in order to achieve a right-hand circularly polarized field. To maintain the resonant condition during the violent acceleration, both period and magnetic field amplitude increase by more than 50% along the axis. We analysed the output energy of the electron beam with a wide energy-acceptance spectrometer. Experimental parameters are summarized in Table 1 . Figure 1: Layout of the helical IFEL experiment at Brookhaven ATF. ( a ) Beamline layout with helical undulator installed just upstream of a wide-angle energy spectrometer shown at the far right. The CO 2 laser beam is injected from the far left-hand side of the beamline while the electron beam is kicked onto the beamline from the left-most dipole. ( b ) Cutaway and zoom of the strongly tapered helical undulator. ( c ) Magnitude of the undulator fields for the high-gradient (orange) and reduced field, high-efficiency (blue) undulator tapering configurations. ( d ) Electron beam trajectories for the high-gradient undulator configuration inferred from the second integrals of the measured fields assuming constant 52 MeV input electron beam energy. The trajectories are superimposed on top of a plot of the 1/ e 2 CO 2 laser spot size as measured by scanning a pyroelectric camera near the waist. Full size image Table 1 Experimental parameters. Full size table Synchronization and timing Picosecond synchronization was achieved by maximizing the IFEL acceleration as the laser pulse was delayed relative to the electron bunch. For this measurement, the electron bunch charge was 100 pC, and its bunch length was 1 ps full-width at half-maximum, which is also the typical linac timing jitter measured at ATF. 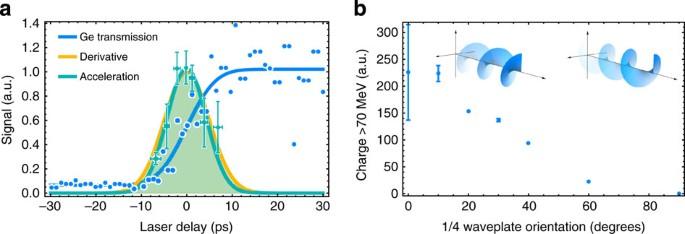Figure 2: Diagnostics. (a) Electron-laser temporal cross-correlation measurements assisted synchronization. Blue points represent relative laser power transmitted through a germanium wafer as the delay between ps-long laser and electron pulses was varied. A standard normal cumulative distribution function fit and its derivative are also displayed yielding an r.m.s. width of 5.0 ps. Maximum IFEL induced energy gains, each scaled by the laser pulse energy, for 30 shots at various delays were binned and displayed in green with error bars showing r.m.s. spread (see Methods). A Gaussian fit to the distribution yielded an r.m.s. width of 4.5 ps. (b) The effect of laser polarization on the interaction was measured. Charge accelerated above 70 MeV is plotted versus quarter waveplate orientation: 0° corresponds to right-handed circularly polarized light, 45° to linear polarization and 90° to left-handed circular polarization. Figure 2a shows both the results of electron beam-controlled transmission through germanium [15] and IFEL energy gain temporal cross-correlation measurements (see Methods). We use this data to infer a root mean square (r.m.s.) laser pulse length of less than 4.5 ps in agreement with spectral width diagnostics and other experiments recently performed at ATF [16] . Assuming 4.5 ps r.m.s. and a 1 mm 1/ e 2 waist, the peak intensity available to drive the IFEL exceeded 2 × 10 13 W cm −2 , which is noticeably lower than that typically used in other laser-driven accelerators. Figure 2: Diagnostics. ( a ) Electron-laser temporal cross-correlation measurements assisted synchronization. Blue points represent relative laser power transmitted through a germanium wafer as the delay between ps-long laser and electron pulses was varied. A standard normal cumulative distribution function fit and its derivative are also displayed yielding an r.m.s. width of 5.0 ps. Maximum IFEL induced energy gains, each scaled by the laser pulse energy, for 30 shots at various delays were binned and displayed in green with error bars showing r.m.s. spread (see Methods). A Gaussian fit to the distribution yielded an r.m.s. width of 4.5 ps. ( b ) The effect of laser polarization on the interaction was measured. Charge accelerated above 70 MeV is plotted versus quarter waveplate orientation: 0° corresponds to right-handed circularly polarized light, 45° to linear polarization and 90° to left-handed circular polarization. Full size image Polarization Another knob to control the strength of the interaction in the helical IFEL is the laser polarization. The interaction of electrons in the helical undulator and elliptically polarized radiation creates two ponderomotive waves with phase velocities given by . For circularly polarized light with the same handedness as the electron motion, only the subluminal wave is present allowing resonant energy transfer. In the experiment, we determined the strength of the coupling by measuring the amount of particles accelerated as a function of laser polarization (see Fig. 2b ). The interaction was maximized (minimized) for matched (opposite) handedness of the laser and undulator polarizations. Reduced interaction was observed for linearly polarized laser light. The accelerated electron spectra were not influenced by the linear polarization angle, showing that the ellipticity of the undulator polarization is negligible. High-gradient acceleration The spectrum for the highest energy laser pulse is shown in Fig. 3 along with spectra from a beam without laser and data from three-dimensional particle tracking simulations [17] (see Methods). The spectrometer image shows a small fraction of the beam accelerated to energies as high as 106 MeV, corresponding to an average accelerating gradient of 100 MeV m −1 —larger than any previous IFEL accelerator and competitive with state-of-the-art high-frequency RF accelerators. Beamline constraints necessitated more relaxed laser focusing, resulting in significantly lower on-axis intensity than design, so that only a small fraction of electrons were accelerated to high energy. During acceleration, electrons dephased at various positions in the undulator where the laser intensity was insufficient to sustain a large enough ponderomotive accelerating gradient to maintain resonance. 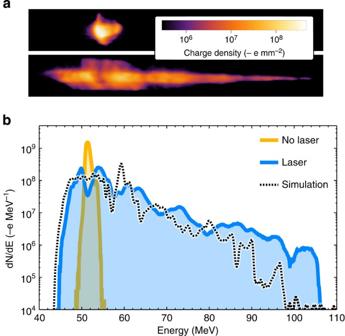Figure 3: Measured electron energy spectra for high-gradient helical IFEL acceleration. (a) Spectrometer images and calibrated spectra with laser-off and laser-on shots for the high-gradient undulator configuration. These images are log-scaled to enhance contrast for parts of the beam with least dispersion. (b) Shown below the images is a log plot of the calibrated spectra with laser-on and -off shots as well as simulation. For this shot, the beam charge and full-width at half-maximum bunch length were 300 pC and 3 ps, respectively, whereas the r.m.s. beam size at the undulator entrance was 400 μm. A small fraction of electrons were accelerated to energies as high as 106 MeV. Figure 3: Measured electron energy spectra for high-gradient helical IFEL acceleration. ( a ) Spectrometer images and calibrated spectra with laser-off and laser-on shots for the high-gradient undulator configuration. These images are log-scaled to enhance contrast for parts of the beam with least dispersion. ( b ) Shown below the images is a log plot of the calibrated spectra with laser-on and -off shots as well as simulation. For this shot, the beam charge and full-width at half-maximum bunch length were 300 pC and 3 ps, respectively, whereas the r.m.s. beam size at the undulator entrance was 400 μm. A small fraction of electrons were accelerated to energies as high as 106 MeV. Full size image High-capture acceleration To improve the quality of the IFEL output beam, the undulator tapering was redesigned to account for the measured focused laser intensity (see Methods). As a result for the ‘high-efficiency’ undulator tapering configuration, we obtained much improved beam spectra with slightly lower final energy. Three representative shots are displayed in Fig. 4 . Up to 30% of the injected beam is accelerated to 93 MeV final energy. A clear monoenergetic bunch of electrons is present with a final output r.m.s. energy spread of 1.8%. The fraction of charge accelerated is large considering that the injected electron bunch was uniformly distributed over many laser periods. Simulations suggest that by prebunching the electron beam at the laser wavelength before injection, the fraction captured could approach unity while increasing peak current considerably (see Supplementary Fig. 2 ). 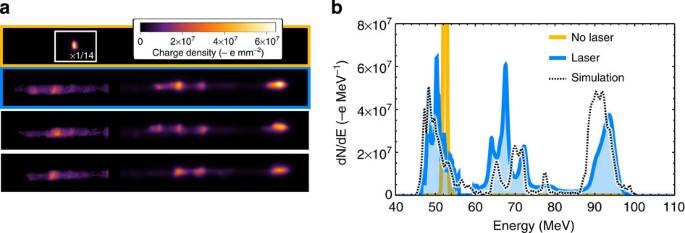Figure 4: Measured electron energy spectra for high-efficiency helical IFEL acceleration. (a) Spectrometer images with calibrated charge density are shown for one laser-off and three representative laser-on shots. The top laser-off shot is scaled by a factor of 1/14 to show its peak intensity. (b) Calibrated spectra (solid) for the first two images and simulation (dashed) are plotted with a linear scale. The input electron beam full-width at half-maximum bunch length was 1 ps, whereas the r.m.s. spot size at the entrance of the undulator was 170 μm. Laser pulse energy for this shot was measured to be 3.7 J, and 26 pC of 110 pC injected was accelerated to a monoenergetic beam with mean energy of 93.5 MeV and 1.8% energy spread. Figure 4: Measured electron energy spectra for high-efficiency helical IFEL acceleration. ( a ) Spectrometer images with calibrated charge density are shown for one laser-off and three representative laser-on shots. The top laser-off shot is scaled by a factor of 1/14 to show its peak intensity. ( b ) Calibrated spectra (solid) for the first two images and simulation (dashed) are plotted with a linear scale. The input electron beam full-width at half-maximum bunch length was 1 ps, whereas the r.m.s. spot size at the entrance of the undulator was 170 μm. Laser pulse energy for this shot was measured to be 3.7 J, and 26 pC of 110 pC injected was accelerated to a monoenergetic beam with mean energy of 93.5 MeV and 1.8% energy spread. Full size image In this second undulator tuning configuration, final energy fluctuations are negligible, reflecting an important advantage of IFEL over other laser-based acceleration schemes in terms of output stability. If the laser provides a sufficient ponderomotive gradient, the IFEL output energy is only set by the tapering of the undulator resonant condition with laser fluctuations at first order only affecting the accelerator capture efficiency. For the shots with laser power above the capture threshold (>180 GW), the energies of the peak charge density of the accelerated beams were normally distributed with a mean of 93.7 MeV and r.m.s. width of 1.2 MeV (<1.3% relative jitter), which is remarkable considering that laser power variation for these shots was 27% r.m.s.. This demonstration also shows that the IFEL output energy could be tuned by controlling the undulator magnetic field. For example, in next generation IFELs, computer control of the magnet gaps or additional small electromagnets throughout the undulator could be used to tune the output energy of the accelerator on demand. Emittance measurement A quadrupole located after the undulator enabled for the first time a measurement of the vertical emittance of the laser-accelerated beam. Because of the rotational symmetry of the helical IFEL interaction and as confirmed by the simulation, it is reasonable to assume that the value obtained also holds for the horizontal plane. 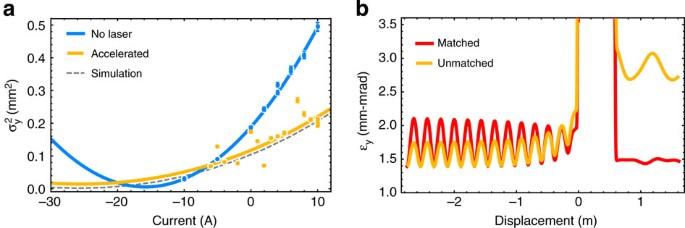Figure 5: Emittance characterization. (a) Scans of vertical spot size versus quadrupole current were used to measure emittances of the unaccelerated and accelerated beams. A fit to the quadrupole scan of the unaccelerated beam yields an emittance of 1.3 mm-mrad in good agreement with a measurement of 1.4 mm-mrad upstream of the experimental setup. The accelerated quadrupole scan yields a measurement of 3 mm-mrad in agreement with simulations (see Methods). (b) Simulations of the experiment show the evolution of the emittance for matched and unmatched beams injected into the 54 cm long undulator positioned at the origin. Emittance oscillations before and after the undulator are due to the electron-laser interaction, whereas the emittance growth within the undulator is a consequence of dispersion as the energy spread of the beam grows. The unmatched beam has an r.m.s. spot size of 170 μm at the undulator’s entrance and an offset of 300 μm, whereas the matched beam is centered with a 80-μm r.m.s. spot size. Particles with energy below 80 MeV are cut from the emittance calculation just after the interaction at 0.6 m. Figure 5a shows the results of the best fits to quad scans [18] for the unaccelerated and accelerated electron beams. The normalized vertical emittance of the unaccelerated beam was measured to be 1.3 mm-mrad in good agreement with measurements upstream of the experimental setup yielding 1.4 mm-mrad. The best fit for normalized vertical emittance yields an estimate of 3 mm-mrad in agreement with the value of 3.3 mm-mrad from the simulations as shown dashed in Fig. 5a . This observed emittance growth is affected by fluctuations in spatial overlap between the electrons, laser and undulator and could be eliminated according to simulations by reducing the e-beam r.m.s. spot size to 80 μm and limiting the relative pointing jitter to <100 μm (see Fig. 5b ). Figure 5: Emittance characterization. ( a ) Scans of vertical spot size versus quadrupole current were used to measure emittances of the unaccelerated and accelerated beams. A fit to the quadrupole scan of the unaccelerated beam yields an emittance of 1.3 mm-mrad in good agreement with a measurement of 1.4 mm-mrad upstream of the experimental setup. The accelerated quadrupole scan yields a measurement of 3 mm-mrad in agreement with simulations (see Methods). ( b ) Simulations of the experiment show the evolution of the emittance for matched and unmatched beams injected into the 54 cm long undulator positioned at the origin. Emittance oscillations before and after the undulator are due to the electron-laser interaction, whereas the emittance growth within the undulator is a consequence of dispersion as the energy spread of the beam grows. The unmatched beam has an r.m.s. spot size of 170 μm at the undulator’s entrance and an offset of 300 μm, whereas the matched beam is centered with a 80-μm r.m.s. spot size. Particles with energy below 80 MeV are cut from the emittance calculation just after the interaction at 0.6 m. Full size image The results of this experiment for the first time demonstrate monoenergetic high-gradient, high-energy gain acceleration of a large fraction of an electron beam injected into a laser-accelerator and suggest the IFEL as an excellent candidate for compact laser-based acceleration in the medium-to-high energy range. Energy gain larger than 50 and 100 MeV m −1 average gradients exceeding those of conventional RF accelerators were obtained using laser intensities of order 10 13 W cm −2 —nearly five orders of magnitude lower than those used with LWFA experiments. By carefully tuning the undulator tapering, we have also demonstrated capture of a large fraction (~30%) of the injected electron beam and monoenergetic acceleration with a final energy spread of the captured beam smaller than 1.8%. Simulations validated by these experimental results show that by using a 20-TW Ti:Sa laser and prebunched beam in a 1-m long IFEL stage, it will be possible to obtain a train of 1 GeV energy bunches of 60 as r.m.s. duration with 0.2% r.m.s. energy spread and >10 kA peak current while preserving excellent output beam quality [19] , enabling applications such as compact laser-accelerator based sources of coherent, sub-femtosecond-scale X-ray pulses with applications in biological and materials research and industrial processing. Experimental setup The 10.3-μm wavelength CO 2 laser beam [13] was reflected by a copper mirror to propagate on the axis of the beamline. A 3-inch diameter NaCl lens with 3.5-m focal length focused the laser beam to a 1/ e 2 spot size (radius) of 1.0 mm near the centre of the undulator. The electron beam [12] injected into the undulator had a mean energy of 52 MeV, charge of 100 pC, bunch length of 1 ps full-width at half-maximum, normalized emittance of 1.4 mm-mrad and an initial energy spread of 0.15%. A quadrupole doublet focused the electron beam to an r.m.s. size of 170 μm at the entrance of the undulator. The undulator was aligned to the beamline axis by minimizing the deflection of a beam propagating along the axis defined by an auxiliary HeNe laser. After exiting the undulator, the electron beam was sent to a dipole-based spectrometer with wide energy acceptance (from 40 to 120 MeV). A quadrupole just before the dipole reduced the beam width in the dispersive plane. The image of the dispersed beam on a scintillator screen was observed via a 45° mirror with a CCD camera. The energy resolution was limited by the betatron beam size at the screen to about 1 MeV. Raw images were acquired with a high-resolution 12-bit camera with a dynamic range wide enough to capture the entire image without saturation, and the images were median filtered and pedestal subtracted to remove noise. The energy was calibrated relative to a dipole current scan with an input beam of fixed energy. Tapered helical undulator The undulator has 11 periods changing from 4.0 cm at the entrance to 5.93 cm at the exit for a total length of 54 cm. The normalized vector potential amplitude varied from 2.0 to 3.9 for the high-gradient undulator field configuration and 2.1 to 3.0 for the high-efficiency configuration. The undulator is the superposition of two Halbach permanent magnet arrays with four pairs of magnets per period per undulator. The blocks are neodymium magnets with a residual magnetization of 1.22 T and cut 33 mm on the major axis and 25 mm on the minor axis with the last 8 mm of the side near the beam linearly tapered from 25 to 12 mm. The gap between magnets for the high-gradient configuration was a constant 15 mm, however, the gap between magnets for the high-efficiency configuration was increased by up to 4.3 mm along the undulator in order to reduce the field strength on axis as shown in Fig. 1c . Properly designed entrance and exit sections maintain the centre of the helical electron trajectories close to the undulator axis. The r.m.s. difference between on-axis fields measured with a hall effect sensor and those calculated with Radia, a three-dimensional magnetostatic simulation [20] , was reduced to less than 1% by finely adjusting the gaps between opposing magnet poles [21] . The helical electron trajectory is calculated by the second integral of the field for a beam energy of 50 MeV and is shown in Fig. 1d . The beam path stays well within the laser waist in order to maximize the field seen by the electrons. Spatial overlap The resonant interaction between laser and electron beam requires spatial and temporal overlap as well as correct-laser polarization. To maintain spatial overlap, entrance and exit magnet arrays kick the electron beam to prevent deflection while the beam rotates in the undulator. The magnetic field was tuned by finely moving undulator magnets to keep the electron trajectories near the undulator axis. The undulator axis was then aligned to the beamline by first using irises attached to the body of the undulator to coalign the entrance and exit to a beamline HeNe laser. Fine tuning was achieved by measuring how the undulator deflected the electron beam and then comparing to the undulator transport matrix to infer offsets, which were then corrected for. During IFEL operation, the beam position was varied about the undulator entrance, and the fraction of electrons captured was observed to decrease for offsets greater than 300 μm. Electron-laser temporal cross-correlation Initial synchronization between electron and laser pulses was obtained by delaying the laser relative to the electron beam so that the separation between a signal from a fast silicon detector on the laser beam path before the undulator and a strip-line located before the input dipole was equal to the time-of-flight distance between them. Finer timing was accomplished by measuring the electron-beam modulated transmission of the laser through a thin germanium plate inserted into the beamline [15] . The laser pulse energy was measured for each shot using a calibrated joulemeter placed to intercept the reflection from a NaCl window. The peak laser power used in this measurement was below threshold for full acceleration so that the IFEL operates in a regime where the induced energy gain of the electrons is proportional to the laser power. As the accelerating gradient is proportional to the laser field amplitude, the maximum energy gain for each shot in Fig. 2a is normalized dividing by the square root of the measured pulse energy to remove the effect of the shot-to-shot laser fluctuations. The resulting curve can be considered a temporal cross-correlation between laser and electron beam based on the IFEL interaction. The 4.5 ps width of the curve is the convolution of the pulse widths of the laser and electron beams as well as their relative time jitter. Laser transport The low-power laser spot size was measured with a pyroelectric camera near the focus and found to follow a Rayleigh range of 30 cm with a beam waist of 1.0 mm and an M 2 of 1.07. The amplified laser pulse spot size was measured by propagating a reflection from the focused laser in air to a waist at the pyroelectric camera with sufficient attenuation to prevent damage and saturation to the sensor. The measured spot size for the amplified pulse was in good agreement (within 6%) with the low-power measurements. Control of the longitudinal and transverse positioning of the laser focus allowed optimization during the experiment. The 3-inch diameter NaCl lens was translated along a rail in order to focus the laser to a waist at various positions along the undulator. The lens was positioned to place the laser waist 7 cm upstream of the undulator midpoint to maximize the accelerator performances as initially suggested by simulation-based optimization and then confirmed experimentally. The maximum laser pulse energy measured upstream of transport was 8 J. Losses during transport reduced the laser power delivered to the undulator. Energy losses from reflections and apertures were measured to be up to 27%, and images of the amplified pulse near the focus indicate that as much as 83% of the energy ended up in the central lobe of the transverse intensity profile because of higher-order transverse modes. Particle tracking simulations The data are compared with three-dimensional particle tracking simulations in the combined laser and undulator fields using all the measured input parameters and field maps (that is, no free parameters). The simulation code [17] solves the Lorentz force equations rather than averaging the motion of the electrons over an undulator period and was previously bench-marked against IFEL experimental results in planar undulators [11] . Tapering configurations The IFEL acceleration experiments were performed using two different undulator tapering configurations. The initial tapering design was designed to be used with the fundamental transverse mode of the CO 2 laser with a 9.6-cm Rayleigh range focused to a peak intensity of 100 TW cm −2 at the undulator midpoint. However, in order to clear a small aperture in the vacuum chamber of the dipole at the entrance to the beamline, the Rayleigh range had to be relaxed to 30 cm, and the laser was only focused to about 20 TW cm −2 . This discrepancy between design and experimental Rayleigh ranges caused a mismatch between the ponderomotive gradient driven by the laser and the gradient in the resonant energy set by the undulator tapering. For a given laser power, the factor of 3 increase in the Rayleigh range implies a reduction in peak on-axis electric field near the undulator midpoint where the resonant energy tapering is steepest. This resulted in reduced capture performance and motivated a retuning of the undulator magnetic field to maximize the fraction of captured electrons. In the second configuration, a gentler field tapering was obtained by slightly increasing the gaps between the permanent magnets to lower the magnetic field amplitude (see blue line in Fig. 1c ). The magnetic field amplitude profile along the undulator was chosen by matching the increase in resonant energy with the available laser-induced ponderomotive gradient [19] and tested with IFEL simulations. The results are excellent evidence of our understanding (theoretical and simulational) of the IFEL physics and the stability of the IFEL process. Quadrupole scan The vertical dimension on the spectrometer screen was used to measure an energy-resolved emittance by quadrupole scan technique [18] varying the current in the short quadrupole magnet positioned just after the undulator (see Fig. 5a ). For the accelerated beam, we calculated the r.m.s. width from a Gaussian fit to the vertical profile of a narrow-energy slice in the dispersive plane at the peak charge density of the accelerated beam (>85 MeV) for the different quadrupole currents. The mean energy of the peak charge density of the accelerated beam was normally distributed with a mean of 93.7 MeV and standard deviation of 1.3%. According to simulations, the emittance growth could in principle be eliminated by reducing the r.m.s. spot size of the electron beam in the undulator by a factor of 2 to 80 μm as shown in Fig. 5b and limiting the relative pointing jitter to less than 100 μm. Experimental uncertainties For the energy measurement, the beam position on the spectrometer screen was recorded with an uncertainty of 70 μm r.m.s., which taking into account the dispersion, and a residual error in the fit for the magnetic field versus current scan yields an error of ±0.04 MeV at 50 MeV to ±0.1 MeV at 90 MeV. Beam position monitors were calibrated by measuring fiducial marks on the screens as well as using a reference known target. Both of these measurements agreed and yielded relative errors of less than 1%. The charge is obtained by recording the measurements of a Faraday cup for 20 shots. A screen charge calibration was obtained summing up the background-subtracted image intensities and correlating the result to the Faraday cup measurement. As both of these measurements are destructive, they were performed successively yielding a charge uncertainty of 8.4%. The CO 2 laser pulse energy was measured during the experiment via a reflection from an NaCl window focused onto a joulemeter and calibrated with high-energy shots relative to another joulemeter placed just before the NaCl window holding vacuum at the entrance of the beamline. How to cite this article: Duris, J. et al. High-quality electron beams from a helical inverse free-electron laser accelerator. Nat. Commun. 5:4928 doi: 10.1038/ncomms5928 (2014).